Oncogenic Ras induces inflammatory cytokine production by upregulating the squamous cell carcinoma antigens SerpinB3/B4 Mounting evidence indicates that oncogenic Ras can modulate cell autonomous inflammatory cytokine production, although the underlying mechanism remains unclear. Here we show that squamous cell carcinoma antigens 1 and 2 (SCCA1/2), members of the Serpin family of serine/cysteine protease inhibitors, are transcriptionally upregulated by oncogenic Ras via MAPK and the ETS family transcription factor PEA3. Increased SCCA expression leads to inhibition of protein turnover, unfolded protein response, activation of NF-κB and is essential for Ras-mediated cytokine production and tumour growth. Analysis of human colorectal and pancreatic tumour samples reveals a positive correlation between Ras mutation, enhanced SCCA expression and IL-6 expression. These results indicate that SCCA is a Ras-responsive factor that plays an important role in Ras-associated cytokine production and tumorigenesis. Constitutively active mutants of Ras are found in a large number of human cancers [1] , [2] . Among the oncogenic activities of mutant Ras, its ability to alter the tumour microenvironment has been well appreciated with numerous studies implicating Ras in various non-cell autonomous processes including basement membrane degradation, immune cell infiltration and angiogenesis [3] , [4] . This tumour microenvironment altering function of Ras is at least partially caused by the ability of Ras to induce the production and secretion of proinflammatory and pro-tumorigenic cytokines. As cellular senescence has been largely attributed to the cytokine secretory response termed senescence-associated secretion phenotype (SASP) [5] , [6] , the possibility remains that oncogene-induced secretory profile is a senescence-independent process on Ras activation. Several reports have implicated Ras in the ability to modulate the tumour microenvironment at least due in part to Ras’ ability to promote the production of cytokines and chemokines such as Interleukin (IL)-6, IL-8, granulocyte–macrophage-colony-stimulating factor (GM-CSF) in a cell autonomous manner [3] , [4] , [7] , [8] . Therefore, it remains to be determined whether premature senescence is a prerequisite of oncogene-induced secretory phenotype, and how Ras mechanistically regulates the expression of the proinflammatory cytokines. Squamous cell carcinoma antigens (SCCAs) are members of the serpin family of endogenous protease inhibitors. Approximately 98 and 92% homologous at their nucleotide and amino-acid levels, respectively, SCCA1 (SerpinB3) and SCCA2 (SerpinB4) are ‘suicide-substrate’ protease inhibitors with differing substrate specificities because of amino-acid differences within their reactive site loop domain [9] . Upregulated in numerous cancers (the cervical, lung, head and neck, liver and breast) [10] , [11] , [12] , [13] , both SCCA1 and SCCA2 are thought to promote cell survival through the inhibition of cell death [14] , [15] . Moreover, the level of SCCA has been shown to predict pathological grade, disease stage, recurrence and response to both radiotherapy and chemotherapy [16] , [17] , [18] . Despite SCCA’s well-reported involvement in cancer, how SCCA is transcriptionally upregulated during transformation and contributes to tumour development remains largely unknown. Here, we study the oncogenic regulation of SCCA and uncover a novel proinflammatory role for SCCA downstream of mutant Ras. We demonstrate that through MAPK signalling and the ETS transcription factor PEA3, oncogenic Ras upregulates the expression of SCCA1/2 (SerpinB3/B4) to promote inflammatory cytokine production and xenograft tumour growth. Moreover, SCCA upregulation is observed in human colorectal and pancreatic cancer. Our findings suggest an important role of serpins in Ras-driven tumorigenesis. Oncogenic Ras upregulates SCCA expression Elevated expression of SCCA has been found in numerous human cancers. However, the underlying molecular mechanism of its upregulation remains unclear. We began to study this by expressing several oncoproteins (HRas V12 , myristolated-Akt (myr-Akt), and c-Myc) in IMR90 primary human lung fibroblasts. While myr-Akt and c-Myc failed to induce SCCA expression, HRas V12 led to a marked increase in SCCA protein levels ( Fig. 1a ). The SCCA antibody utilized was unable to distinguish between the SCCA isoforms [10] , although quantitative reverse-transcription PCR (qRT–PCR) analysis revealed an increase in the transcript levels of both SCCA1 and SCCA2 in response to Ras V12 expression ( Fig. 1b ). This is not surprising as the two SCCA isoforms are tandemly arranged on human chromosome 18q and their promoters are highly homologous [19] . 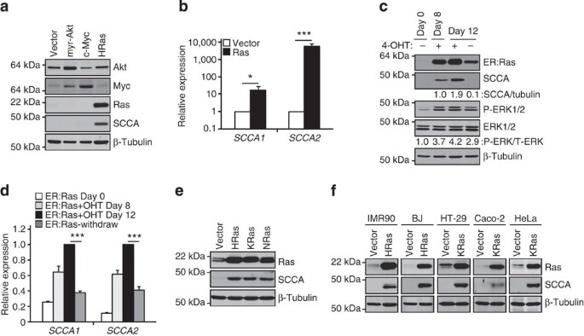Figure 1: Oncogenic Ras upregulates SCCA expression. (a) Indicated oncogenes were stably expressed in IMR90 cells. Whole-cell lysates were obtained and analysed by western blot with indicated antibodies. (b) Total RNA was extracted from vector-control or RasV12-expressing IMR90 cells. SCCA1 and SCCA2 transcript levels were analysed via qRT–PCR and normalized to that in vector-control cells. Data shown are mean+s.e.m. of three independent experiments performed in triplicate. (c,d) IMR90 cells expressing the ER:RasV12fusion protein were treated with 4-OHT for 8 days, split and either cultured in media containing 4-OHT or withdrew 4-OHT for additional 4 days. (c) Whole-cell lysates were analysed by western blot with indicated antibodies. (d) Total RNA was extracted, and SCCA1 and SCCA2 transcript levels were analysed via qRT–PCR, and normalized to that of Day 12 ER:Ras with 4-OHT cells. Data shown are mean+s.e.m. of three independent experiments performed in triplicate. (e) Indicated oncogenic Ras proteins were stably expressed in IMR90 cells. Whole-cell lysates were obtained and analysed by western blot with indicated antibodies. (f) HRasV12was stably expressed in IMR90 and BJ cell lines. KRasV12was stably expressed in HT-29, Caco-2 and HeLa cells. Whole-cell lysates were obtained and analysed by western blot with indicated antibodies. *P<0.05; ***P<0.001 byt-test. Figure 1: Oncogenic Ras upregulates SCCA expression. ( a ) Indicated oncogenes were stably expressed in IMR90 cells. Whole-cell lysates were obtained and analysed by western blot with indicated antibodies. ( b ) Total RNA was extracted from vector-control or Ras V12 -expressing IMR90 cells. SCCA1 and SCCA2 transcript levels were analysed via qRT–PCR and normalized to that in vector-control cells. Data shown are mean+s.e.m. of three independent experiments performed in triplicate. ( c , d ) IMR90 cells expressing the ER:Ras V12 fusion protein were treated with 4-OHT for 8 days, split and either cultured in media containing 4-OHT or withdrew 4-OHT for additional 4 days. ( c ) Whole-cell lysates were analysed by western blot with indicated antibodies. ( d ) Total RNA was extracted, and SCCA1 and SCCA2 transcript levels were analysed via qRT–PCR, and normalized to that of Day 12 ER:Ras with 4-OHT cells. Data shown are mean+s.e.m. of three independent experiments performed in triplicate. ( e ) Indicated oncogenic Ras proteins were stably expressed in IMR90 cells. Whole-cell lysates were obtained and analysed by western blot with indicated antibodies. ( f ) HRas V12 was stably expressed in IMR90 and BJ cell lines. KRas V12 was stably expressed in HT-29, Caco-2 and HeLa cells. Whole-cell lysates were obtained and analysed by western blot with indicated antibodies. * P <0.05; *** P <0.001 by t -test. Full size image To determine whether persistent Ras signalling is required for SCCA expression, we used the oestrogen receptor (ER):Ras V12 fusion protein that allows for Ras V12 stabilization on the addition of 4-hydroxytamoxifen (4-OHT) to the culture medium [20] . While 4-OHT induced the expression of Ras and SCCA ( Fig. 1c ), removal of 4-OHT led to a drastic reduction in Ras V12 protein levels and diminished downstream signalling indicated by decreased phospho-ERK, accompanied by a reduction of SCCA at both protein and transcript levels ( Fig. 1c,d ), indicating that sustained Ras signalling is required for maintaining SCCA expression. In addition to HRas V12 , expression of KRas V12 or NRas Q61 also resulted in elevated SCCA expression in IMR90 cells ( Fig. 1e ). Similar to IMR90 cells, increased SCCA expression was observed by expressing HRas V12 in the BJ primary human foreskin fibroblast cells, and by expression of KRas V12 in a number of cancer cell lines with wild-type Ras, including the colon cancer cell lines HT-29 and Caco-2, and HeLa cells ( Fig. 1f ). Taken together, these results indicate that upregulation of SCCA expression is a general feature of oncogenic Ras proteins in various human cell lines. It is important to note that in IMR90 and BJ fibroblasts expression of Ras V12 elicits oncogene-induced senescence [21] . The upregulation of SCCA in response to Ras V12 in Caco-2, HT-29 and HeLa cells, which do not undergo senescence [3] , [22] , suggests that upregulation of SCCA by Ras V12 is independent of cellular senescence. To further elucidate that the increased SCCA expression is not a consequence of cellular senescence, we induced premature senescence by treating IMR90 cells with etoposide or H 2 O 2 and replicative senescence by continually passaging the cells. Indeed, unlike Ras V12 , these senescence-inducing conditions failed to upregulate SCCA expression ( Fig. 2 ). These results indicate that expression of oncogenic Ras stimulates expression of SCCA in a manner that is independent of oncogene-induced senescence. 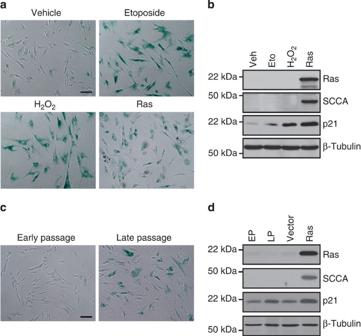Figure 2: DNA damage-induced and replicative senescence fails to upregulate SCCA. (a,b) IMR90 cells were treated with vehicle-control, etoposide (10 μM) for 48 h, H2O2(10 μM) for 1 h, or stably transduced with HRasV12, then analysed 7 days post-treatment. (a) Cells were stained for β-Gal activity. Representative images are shown. (b) Whole-cell lysates were analysed by western blot with indicated antibodies. (c,d) IMR90 cells were continuously passaged and harvested at passage 15 as early passage (EP) or at passage 30 as late passage. (c) Cells were stained for β-galactosidase activity. Representative images are shown. (d) Whole-cell lysates were analysed by western blot with indicated antibodies. Note that while all the conditions induce cellular senescence, only RasV12led to SCCA expression. Scale bar=100 μm. Figure 2: DNA damage-induced and replicative senescence fails to upregulate SCCA. ( a , b ) IMR90 cells were treated with vehicle-control, etoposide (10 μM) for 48 h, H 2 O 2 (10 μM) for 1 h, or stably transduced with HRas V12 , then analysed 7 days post-treatment. ( a ) Cells were stained for β-Gal activity. Representative images are shown. ( b ) Whole-cell lysates were analysed by western blot with indicated antibodies. ( c , d ) IMR90 cells were continuously passaged and harvested at passage 15 as early passage (EP) or at passage 30 as late passage. ( c ) Cells were stained for β-galactosidase activity. Representative images are shown. ( d ) Whole-cell lysates were analysed by western blot with indicated antibodies. Note that while all the conditions induce cellular senescence, only Ras V12 led to SCCA expression. Scale bar=100 μm. Full size image Ras-induced SCCA is dependent on the MAPK/PEA3 pathway To elucidate the mechanism by which Ras V12 stimulates SCCA expression, we used pharmacological inhibitors to selectively inhibit MAPK and Akt pathways that are well characterized to be activated by Ras [2] , [23] . While inhibition of Akt signalling had little to no effect on SCCA expression ( Fig. 3a,b ), the MEK inhibitor U0126 caused a marked inhibition of both SCCA1 and SCCA2 transcription in both IMR90 ( Fig. 3c,d ) and HeLa cells ( Supplementary Fig. 1a,b ). Similarly, expression of the dominant-negative ERK2 blocked Ras-induced SCCA expression ( Supplementary Fig. 1c,d ). Along the Ras/Raf/MAPK/ERK pathway, expression of oncogenic BRaf V600E also induced SCCA expression ( Supplementary Fig. 1e ). We next sought to identify which transcription factor may be mediating Ras-induced expression of SCCA. The ETS transcription factor family member PEA3 has been shown to be modulated by MAPK via sumolyation [24] and can activate SCCA transcription [25] . Indeed, silencing of PEA3 in Ras V12 -expressing cells ( Fig. 3e ) resulted in a drastic decrease of both SCCA1 and SCCA2 at protein and transcript levels ( Fig. 3f,g ), without affecting MAPK signalling indicated by similar levels of phospho-ERK in Ras V12 -expressing cells ( Fig. 3f ). This PEA3-dependent SCCA expression was also observed in Ras V12 -expressing HeLa cells ( Supplementary Fig. 2a–c ) and was rescued by expression of wild-type murine PEA3, but not by a PEA3 sumolyation-defective mutant [24] ( Supplementary Fig. 2d–f ). These results indicate that mutant Ras leads to SCCA upregulation via the MAPK/PEA3 pathway. 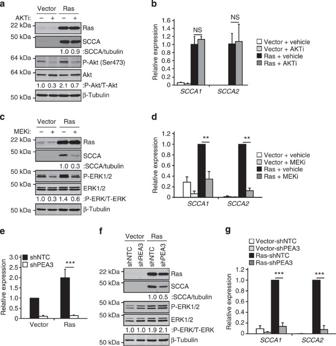Figure 3: SCCA upregulation is mediated by MAPK/PEA3. (a,b) Vector-control or HRasV12-expressing IMR90 cells were treated with either vehicle-control or AKTi (10 μM) for 24 h. (a) Whole-cell lysates were analysed by western blot with indicated antibodies. (b) Total RNA was extracted and SCCA1 and SCCA2 transcript levels were analysed via qRT–PCR, and normalized to RasV12cells treated with vehicle-control. Data shown are mean+s.e.m. of two independent experiments performed in triplicate. (c,d) Vector-control or HRasV12-expressing IMR90 cells were treated with either vehicle-control (DMSO) or U1026 (MEKi, 10 μM) for 24 h. (c) Whole-cell lysates were analysed by western blot with indicated antibodies. (d) Total RNA was extracted, and SCCA1 and SCCA2 transcript levels were analysed via qRT–PCR and normalized to that of Ras-expressing cells treated with vehicle. Data shown are mean+s.e.m. of three independent experiments performed in triplicate. (e–g) Vector-control or HRasV12-expressing IMR90 cells were stably infected with lentiviral shNTC (non-target control) or shPEA3. (e) Successful silencing of PEA3 was confirmed via qRT–PCR and normalized to that in vector-control cells with shNTC. Data shown are mean+s.e.m. of three independent experiments performed in triplicate. (f) Whole-cell lysates were analysed through western blot with indicated antibodies. (g) Total RNA was analysed for the transcript levels of SCCA1 and SCCA2 via qRT–PCR and normalized to that in Ras-expressing cells with shNTC. Data shown are mean+s.e.m. of three independent experiments performed in triplicate. **P<0.01; ***P<0.001; NS, non-significant byt-test. Figure 3: SCCA upregulation is mediated by MAPK/PEA3. ( a , b ) Vector-control or HRas V12 -expressing IMR90 cells were treated with either vehicle-control or AKTi (10 μM) for 24 h. ( a ) Whole-cell lysates were analysed by western blot with indicated antibodies. ( b ) Total RNA was extracted and SCCA1 and SCCA2 transcript levels were analysed via qRT–PCR, and normalized to Ras V12 cells treated with vehicle-control. Data shown are mean+s.e.m. of two independent experiments performed in triplicate. ( c , d ) Vector-control or HRas V12 -expressing IMR90 cells were treated with either vehicle-control (DMSO) or U1026 (MEKi, 10 μM) for 24 h. ( c ) Whole-cell lysates were analysed by western blot with indicated antibodies. ( d ) Total RNA was extracted, and SCCA1 and SCCA2 transcript levels were analysed via qRT–PCR and normalized to that of Ras-expressing cells treated with vehicle. Data shown are mean+s.e.m. of three independent experiments performed in triplicate. ( e – g ) Vector-control or HRas V12 -expressing IMR90 cells were stably infected with lentiviral shNTC (non-target control) or shPEA3. ( e ) Successful silencing of PEA3 was confirmed via qRT–PCR and normalized to that in vector-control cells with shNTC. Data shown are mean+s.e.m. of three independent experiments performed in triplicate. ( f ) Whole-cell lysates were analysed through western blot with indicated antibodies. ( g ) Total RNA was analysed for the transcript levels of SCCA1 and SCCA2 via qRT–PCR and normalized to that in Ras-expressing cells with shNTC. Data shown are mean+s.e.m. of three independent experiments performed in triplicate. ** P <0.01; *** P <0.001; NS, non-significant by t -test. Full size image SCCA is essential for Ras-induced cytokine production Next we examined the biological role of elevated SCCA expression. We chose to focus on using the IMR90 cell line that is widely used for studying the effect of Ras activation during the early phase of tumorigenesis. We began by examining the downstream signalling pathways activated by oncogenic Ras (MAPK, Akt, NF-κB). To this end, SCCA expression was silenced in Ras V12 -expressing cells using two independent shRNA constructs that effectively silenced both SCCA1 and SCCA2 ( Fig. 4a ), and the signalling pathways examined by respective phosphorylation antibodies. While loss of SCCA had little to no effect on the ability of mutant Ras to activate Akt and MAPK phosphorylation ( Fig. 4b ), loss of SCCA significantly diminished Ras V12 -induced RelA/p65 phosphorylation that is indicative of NF-κB activation ( Fig. 4b ). This effect was further confirmed by utilizing a NF-κB luciferase reporter construct ( Fig. 4c ). 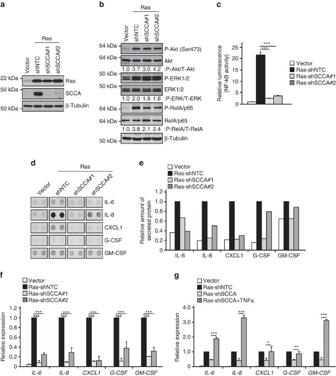Figure 4: SCCA modulates Ras-induced cytokine production. (a–f) Vector-control or HRasV12-expressing IMR90 cells were stably infected with lentiviral shRNA control (shNTC) or two independent hairpins targeting SCCA. (a,b) Whole-cell lysates were analysed by western blot with indicated antibodies. (c) Cells were transfected with an NF-κB luciferase reporter and a renilla luciferase construct. Twenty-four hours post transfection, cells were lysed and luminescence was quantified. NF-κB luciferase activity was standardized based on renilla luciferase activity and normalized to that of vector-control cells. Data shown are mean+s.e.m. of three independent experiments performed in triplicate. (d) Culture media were collected and subjected to a cytokine antibody array. The representative of two independent blots of indicated cytokines are shown. (e) The relative amount of cytokines was quantified and normalized to that of RasV12-shNTC cells. (f) Total RNA was extracted and cytokine transcript levels were analysed via qRT–PCR, and normalized to that of RasV12-shNTC cells. Data shown are mean+s.e.m. of three independent experiments performed in triplicate. (g) Ras-shSCCA cells were treated with TNFα (50 ng μl−1) for 16 h. Total RNA was extracted and cytokine transcript levels were analysed via qRT–PCR and normalized to that of RasV12-shNTC cells. Data shown are mean+s.e.m. of two independent experiments performed in triplicate. *P<0.05; **P<0.01; ***P<0.001 byt-test. Figure 4: SCCA modulates Ras-induced cytokine production. ( a – f ) Vector-control or HRas V12 -expressing IMR90 cells were stably infected with lentiviral shRNA control (shNTC) or two independent hairpins targeting SCCA. ( a , b ) Whole-cell lysates were analysed by western blot with indicated antibodies. ( c ) Cells were transfected with an NF-κB luciferase reporter and a renilla luciferase construct. Twenty-four hours post transfection, cells were lysed and luminescence was quantified. NF-κB luciferase activity was standardized based on renilla luciferase activity and normalized to that of vector-control cells. Data shown are mean+s.e.m. of three independent experiments performed in triplicate. ( d ) Culture media were collected and subjected to a cytokine antibody array. The representative of two independent blots of indicated cytokines are shown. ( e ) The relative amount of cytokines was quantified and normalized to that of Ras V12 -shNTC cells. ( f ) Total RNA was extracted and cytokine transcript levels were analysed via qRT–PCR, and normalized to that of Ras V12 -shNTC cells. Data shown are mean+s.e.m. of three independent experiments performed in triplicate. ( g ) Ras-shSCCA cells were treated with TNFα (50 ng μl −1 ) for 16 h. Total RNA was extracted and cytokine transcript levels were analysed via qRT–PCR and normalized to that of Ras V12 -shNTC cells. Data shown are mean+s.e.m. of two independent experiments performed in triplicate. * P <0.05; ** P <0.01; *** P <0.001 by t -test. Full size image Activation of NF-κB signalling has been attributed to cytokine production downstream of Ras activation [26] . Indeed, inhibition of NF-κB signalling using the pharmacological inhibitor BAY11-7082 abrogated Ras-induced cytokine production in IMR90 and HeLa cells ( Supplementary Fig. 3 ). Therefore, we examined whether SCCA plays a role in Ras-induced cytokine production and performed a quantitative cytokine array analysis using cell culture media. In agreement with literature [5] , [6] , Ras V12 -expressing cells displayed a marked increase in a spectrum of cytokines including IL-6, IL-8, CXCL1, G-CSF and GM-CSF ( Fig. 4d ). Consistent with the observed decrease in NF-κB signalling ( Fig. 4b,c ), this increased cytokine expression was significantly abrogated on SCCA silencing ( Fig. 4d,e ). Quantitative RT-PCR analysis revealed that the suppression of cytokine production was due to transcriptional downregulation ( Fig. 4f ) and was rescued by ectopically activating NF-κB signalling with TNFα treatment ( Fig. 4g ). The SCCA-dependent NF-κB activation and cytokine production downstream of oncogenic Ras were also observed in HeLa and Caco-2 cells ( Supplementary Fig. 4 ). The introduction of oncogenic Ras in IMR90 elicits a DNA damage response that has been reported to mediate cytokine production [6] , [27] . However, silencing of SCCA had virtually no effect on Ras-induced DNA damage indicated by the phosphorylation of H2A.X ( Fig. 5a,b ) or the senescence-associated cell cycle arrest ( Fig. 5c ). Taken together, these results indicate that SCCA plays an essential role in Ras-mediated NF-κB activation and inflammatory cytokine production that is independent of the DNA-damage response. 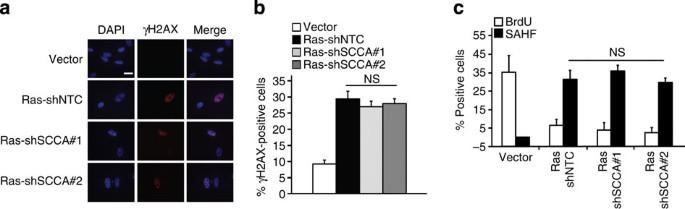Figure 5: Silencing of SCCA does not interfere with the DNA-damage response. (a–c) Vector-control or HRasV12-expressing IMR90 cells were stably infected with lentiviral shRNA control (shNTC) or two independent hairpins targeting SCCA (same cells as shown inFig. 4). (a) Immunofluorescence against γH2A.X was performed. Representative images are shown; scale bar, 20 μm. (b) Quantification of percent γH2A.X-positive cells is shown. Note that silencing of SCCA does not compromise Ras-induced DNA damage. Data shown are mean+s.e.m. of three independent experiments. (c) Cells were cultured with BrdU (10 μM) for 6 h and immunofluorescence against BrdU was performed. Quantification of BrdU-positive and senescence-associated heterochromatic foci (SAHF)-positive cells are shown. Data shown are mean+s.e.m. of three independent experiments. NS, non-significant byt-test. Figure 5: Silencing of SCCA does not interfere with the DNA-damage response. ( a – c ) Vector-control or HRas V12 -expressing IMR90 cells were stably infected with lentiviral shRNA control (shNTC) or two independent hairpins targeting SCCA (same cells as shown in Fig. 4 ). ( a ) Immunofluorescence against γH2A.X was performed. Representative images are shown; scale bar, 20 μm. ( b ) Quantification of percent γH2A.X-positive cells is shown. Note that silencing of SCCA does not compromise Ras-induced DNA damage. Data shown are mean+s.e.m. of three independent experiments. ( c ) Cells were cultured with BrdU (10 μM) for 6 h and immunofluorescence against BrdU was performed. Quantification of BrdU-positive and senescence-associated heterochromatic foci (SAHF)-positive cells are shown. Data shown are mean+s.e.m. of three independent experiments. NS, non-significant by t -test. Full size image SCCA promotes cytokine production by inducing the unfolded protein response We next sought to understand how SCCA promotes Ras-mediated NF-κB activation and cytokine production. A possible mechanism is through upregulation of the unfolded protein response (UPR), which has been implicated in mediating NF-κB activation and inflammatory transcriptional programmes [28] . Our previous work showed that SCCA leads to decreased lysosomal and proteasomal protein turnover, two major protein degradation pathways, and hence increases the steady-state level of ER stress [29] . Thus, we speculated that mutant Ras induces ER stress through upregulation of SCCA. Indeed, the ability of Ras V12 to promote an ER stress response has been reported [30] . Silencing of SCCA relieved the Ras-induced inhibition of protein turnover as measured through total ubiquitinated proteins ( Fig. 6a ). Furthermore, while Ras V12 cells showed a robust increase in UPR indicated by the appearance of proteolytically cleaved ATF6 as well as both unspliced and spliced XBP1, this response was significantly reduced in SCCA-silenced cells ( Fig. 6b ), indicating that SCCA mediates the UPR induced by Ras V12 . Silencing of ATF6 or XBP1 in Ras V12 -expressing cells ( Fig. 6c ) drastically diminished Ras V12 -induced cytokine production ( Fig. 6d–f ; Supplementary Fig. 5 ) that was accompanied by decreased RelA/p65 phosphorylation ( Fig. 6g ; Supplementary Fig. 5 ). Conversely, ectopic expression of the transcriptionally active spliced variant of XBP1 (XBP1s) restored cytokine production in Ras V12 cells when SCCA was silenced ( Fig. 6h,i ). These results indicate that SCCA modulates cytokine production downstream of mutant Ras by stimulating UPR. 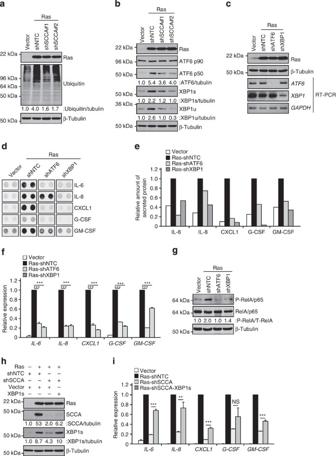Figure 6: SCCA promotes cytokine production by inducing UPR. (a,b) Vector-control or HRasV12-expressing IMR90 cells were stably infected with lentiviral shRNA control (shNTC) or two independent hairpins targeting SCCA. Whole-cell lysates were analysed by western blot with indicated antibodies. Quantification of the ubiquitin blot inawas performed by Image J using the full-length of each lane. (c–g) Vector-control or HRasV12IMR90 cells were stably infected with lentiviral shRNA control (shNTC) or shRNA hairpins targeting ATF6 or XBP1. (c,g) Whole-cell lysates were analysed by western blot with indicated antibodies. (d) Culture media were collected and subjected to a cytokine antibody array. The blots of indicated cytokines are shown. (e) The relative amount of cytokines was quantified and normalized to that of RasV12-shNTC cells. (f) Total RNA was extracted and cytokine transcript levels were analysed via qRT–PCR and normalized against that in RasV12-shNTC cells. Data shown are mean+s.e.m. of three independent experiments performed in triplicate. (h,i) Vector-control or HRasV12IMR90 cells were stably infected with lentiviral shRNA control (shNTC) or shSCCA, together with vector-control or XBP1s-expressing construct. (h) Whole-cell lysates were analysed by western blot with indicated antibodies. (i) Total RNA was extracted and cytokine transcript levels were analysed via qRT–PCR and normalized against that in RasV12-shNTC cells. Data shown are mean+s.e.m. of three independent experiments performed in triplicate. **P<0.01; ***P<0.001; NS, non-significant byt-test. Figure 6: SCCA promotes cytokine production by inducing UPR. ( a , b ) Vector-control or HRas V12 -expressing IMR90 cells were stably infected with lentiviral shRNA control (shNTC) or two independent hairpins targeting SCCA. Whole-cell lysates were analysed by western blot with indicated antibodies. Quantification of the ubiquitin blot in a was performed by Image J using the full-length of each lane. ( c – g ) Vector-control or HRas V12 IMR90 cells were stably infected with lentiviral shRNA control (shNTC) or shRNA hairpins targeting ATF6 or XBP1. ( c , g ) Whole-cell lysates were analysed by western blot with indicated antibodies. ( d ) Culture media were collected and subjected to a cytokine antibody array. The blots of indicated cytokines are shown. ( e ) The relative amount of cytokines was quantified and normalized to that of Ras V12 -shNTC cells. ( f ) Total RNA was extracted and cytokine transcript levels were analysed via qRT–PCR and normalized against that in Ras V12 -shNTC cells. Data shown are mean+s.e.m. of three independent experiments performed in triplicate. ( h , i ) Vector-control or HRas V12 IMR90 cells were stably infected with lentiviral shRNA control (shNTC) or shSCCA, together with vector-control or XBP1s-expressing construct. ( h ) Whole-cell lysates were analysed by western blot with indicated antibodies. ( i ) Total RNA was extracted and cytokine transcript levels were analysed via qRT–PCR and normalized against that in Ras V12 -shNTC cells. Data shown are mean+s.e.m. of three independent experiments performed in triplicate. ** P <0.01; *** P <0.001; NS, non-significant by t -test. Full size image SCCA is upregulated in colorectal and pancreatic cancers Our results thus far show that SCCA is a Ras-responsive gene that plays an essential role in Ras-induced cytokine production. We next sought to identify an in vivo connection between Ras and SCCA expression. Using TCGA (The Cancer Genome Atlas) data of human colorectal cancer, which were available with sizeable samples with the KRas mutation, we identified a positive correlation between the presence of mutant Ras and SCCA upregulation ( Fig. 7a ). We also chose to examine pancreatic ductal adenocarcinoma (PDAC), where the mutant KRas functions as the primary driver [31] . It also offers a unique model where the precursor lesions to PDAC have a defined pathological progression [31] . To this end, we analysed the pancreatic cancer gene expression data sets for SCCA expression through Oncomine. In the seven available patient data sets, SCCA1 mRNA was upregulated in six and SCCA2 mRNA in three independent data sets [32] , [33] , [34] , [35] , [36] , [37] ( Fig. 7b–d ). Of note, the Logsdon data set [37] identified both SCCA1 and SCCA2 to be upregulated in pancreatic cancer when compared with chronic pancreatitis ( Fig. 7d ). To further examine the association of SCCA expression in human pancreatic cancer, we performed immunohistochemistry (IHC) for SCCA using a pancreatic cancer tissue microarray. While all non-neoplastic/normal pancreatic samples were negative for SCCA expression, positive staining for SCCA was seen throughout all stages of pancreatic cancer progression. The incidence of SCCA positivity increased in relation to the progression of pancreatic cancer: 2 out of 17 (11.8%) PanIN-1 lesions, 5 out of 19 (26.3%) PanIN-2 lesions, 8 out of 15 (53.3%) PanIN-3 lesions and 20 out of 30 (66.7%) of PDAC ( Fig. 7e ; P <0.001). Moreover, consistent with the result that SCCA promotes inflammatory cytokine production in cultured cells, IHC of IL-6 on the same panel of pancreatic tissues showed a positive correlation between IL-6 and SCCA in both PDAC ( Fig. 7f,g ) and PanIN ( Supplementary Fig. 6 ) samples. 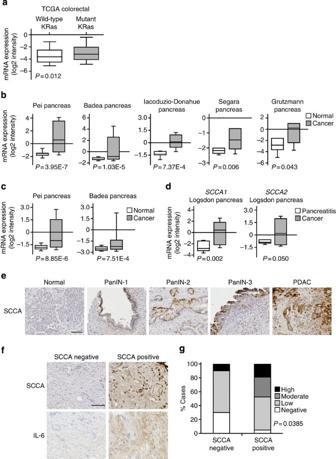Figure 7: SCCA is upregulated in human colorectal and pancreatic cancer. (a) TCGA human colorectal cancer data of somatic mutation and RNA expression from Broad Institute’s Genome Data Analysis Center were analysed. There were 207 human colorectal tumours that have both somatic mutation and mRNA expression data available. KRas was mutated in 87 out of the 207 samples. By comparing SCCA mRNA expression level of the groups with wild-type and mutated KRas, SCCA expression was found to be significantly higher in the group with KRas mutation. Boxplots with whisker from 10 to 90 percentile are shown. SCCA expression log2 intensity values for wild-type (n=120) and mutant (n=87) KRas samples are shown.P=0.012 by Wilcoxon Rank Sum test. (b–d) Oncomine (www.oncomine.org) data sets were analysed for SCCA1 (b) or SCCA2 (c) mRNA expression levels in normal pancreatic tissue and pancreatic cancer, or for SCCA1 and SCCA2 mRNA expression levels in chronic pancreatitis and pancreatic cancer (d). The boxes represent the interquartile range. Whiskers represent the 10th–90th percentile range. Bars represent the median.P-values were calculated by two-samplet-test. (e–g) IHC against SCCA and IL-6 was performed on the corresponding serial pancreatic tissue microarrays. (e) Representative images of normal pancreatic tissue and SCCA-positive PanIN 1, PanIN-2, PanIN-3 and PDAC samples are shown; scale bar, 100 μm. (f) Representative images of SCCA/IL-6-negative and SCCA/IL-6-positive grade III PDAC samples; scale bar, 50 μm. (g) Quantification of IL-6 staining in SCCA-negative and SCCA-positive samples.χ2-test for trend was used to determine significance,P=0.0385. Figure 7: SCCA is upregulated in human colorectal and pancreatic cancer. ( a ) TCGA human colorectal cancer data of somatic mutation and RNA expression from Broad Institute’s Genome Data Analysis Center were analysed. There were 207 human colorectal tumours that have both somatic mutation and mRNA expression data available. KRas was mutated in 87 out of the 207 samples. By comparing SCCA mRNA expression level of the groups with wild-type and mutated KRas, SCCA expression was found to be significantly higher in the group with KRas mutation. Boxplots with whisker from 10 to 90 percentile are shown. SCCA expression log2 intensity values for wild-type ( n =120) and mutant ( n =87) KRas samples are shown. P =0.012 by Wilcoxon Rank Sum test. ( b – d ) Oncomine ( www.oncomine.org ) data sets were analysed for SCCA1 ( b ) or SCCA2 ( c ) mRNA expression levels in normal pancreatic tissue and pancreatic cancer, or for SCCA1 and SCCA2 mRNA expression levels in chronic pancreatitis and pancreatic cancer ( d ). The boxes represent the interquartile range. Whiskers represent the 10th–90th percentile range. Bars represent the median. P -values were calculated by two-sample t -test. ( e – g ) IHC against SCCA and IL-6 was performed on the corresponding serial pancreatic tissue microarrays. ( e ) Representative images of normal pancreatic tissue and SCCA-positive PanIN 1, PanIN-2, PanIN-3 and PDAC samples are shown; scale bar, 100 μm. ( f ) Representative images of SCCA/IL-6-negative and SCCA/IL-6-positive grade III PDAC samples; scale bar, 50 μm. ( g ) Quantification of IL-6 staining in SCCA-negative and SCCA-positive samples. χ 2 -test for trend was used to determine significance, P =0.0385. Full size image Endogenous SCCA promotes IL-6 production and tumorigenesis To further explore the physiological relevance of SCCA, we tested the expression and function of SCCA in a setting when mutant Ras is expressed at endogenous levels. Ras V12 failed to induce the expression of the SCCA paralogues Serpinb3a or Serpinb3b in immortalized MEF NIH3T3 ( Supplementary Fig. 7a ) or in primary MEFs ( Supplementary Fig. 7b ). The failure to detect upregulation of SCCA paralogues in the murine system prevented us from using the well-established LSL-KRas mouse model [38] . Hence, we instead examined a panel of human pancreatic cancer cell lines that harbour the mutant KRas. We found five out of nine cell lines to be positive for SCCA expression ( Fig. 8a ). In the cell lines that displayed detectable levels of SCCA and can tolerate loss of KRas (CFPAC-1, L3.6 and Capan-1), silencing of mutant KRas significantly reduced SCCA expression ( Fig. 8b ). Consistent with the essential role of SCCA in Ras-mediated cytokine production, silencing of SCCA in three SCCA-positive cell lines resulted in decreased expression of IL-6, whereas the SCCA shRNAs did not affect IL-6 expression in the SCCA-low PANC-1 cells ( Fig. 8c ). Moreover, while silencing of SCCA in CFPAC-1, L3.6 and HPAF-II cells did not compromise cell proliferation in cell culture ( Supplementary Fig. 8 ), it led to impaired xenograft tumour growth in all three cell lines ( Fig. 8d ). These results, taken together with the above finding that SCCA positivity correlates with progression of pancreatic cancer development ( Fig. 7e ), indicate that SCCA expression is under the control of mutant Ras expressed at endogenous level, and that the SCCA-mediated inflammatory response plays a pro-tumorigenic role in Ras-driven cancer. 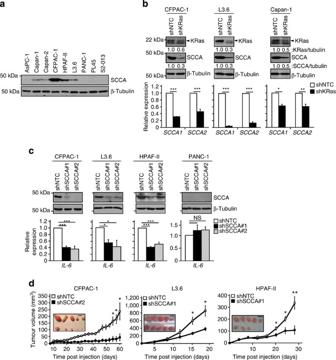Figure 8: Ras-dependent SCCA expression promotes IL-6 production and tumorigenesis in human pancreatic cancer cell lines. (a) Whole-cell lysates from a panel of pancreatic cancer cells were obtained and analysed through western blot with indicated antibodies. (b) Indicated cell lines were stably infected with lentiviral shNTC or shKRas. Whole-cell lysates were analysed through western blot with indicated antibodies. Note that the Ras antibody utilized is a pan-Ras antibody and KRas is indicated by arrowhead. Total RNA was extracted, and SCCA1 and SCCA2 transcript levels were analysed via qRT–PCR and normalized to that of shNTC cells. Data shown are mean+s.e.m. of three independent experiments performed in triplicate. (c) Indicated cell lines were stably infected with lentiviral shNTC or shSCCA. Whole-cells lysates were analysed through western blot with indicated antibodies. Total RNA was extracted and IL-6 transcript levels were analysed via qRT–PCR. Data shown are mean+s.e.m. of three independent experiments performed in triplicate. Relative level of transcript was normalized to that of shNTC cells. Note that silencing of SCCA in PANC-1 cells, which have undetectable SCCA expression, had virtually no effect on IL-6 production. (d) CFPAC-1, L3.6 and HPAF-II cells were injected into the flanks of athymic nude mice and monitored for tumour growth;n=5. Representative images of tumour and the tumour growth curve±s.e.m. are shown; scale bar, 1 cm. *P<0.05, **P<0.01, ***P<0.001 byt-test. Figure 8: Ras-dependent SCCA expression promotes IL-6 production and tumorigenesis in human pancreatic cancer cell lines. ( a ) Whole-cell lysates from a panel of pancreatic cancer cells were obtained and analysed through western blot with indicated antibodies. ( b ) Indicated cell lines were stably infected with lentiviral shNTC or shKRas. Whole-cell lysates were analysed through western blot with indicated antibodies. Note that the Ras antibody utilized is a pan-Ras antibody and KRas is indicated by arrowhead. Total RNA was extracted, and SCCA1 and SCCA2 transcript levels were analysed via qRT–PCR and normalized to that of shNTC cells. Data shown are mean+s.e.m. of three independent experiments performed in triplicate. ( c ) Indicated cell lines were stably infected with lentiviral shNTC or shSCCA. Whole-cells lysates were analysed through western blot with indicated antibodies. Total RNA was extracted and IL-6 transcript levels were analysed via qRT–PCR. Data shown are mean+s.e.m. of three independent experiments performed in triplicate. Relative level of transcript was normalized to that of shNTC cells. Note that silencing of SCCA in PANC-1 cells, which have undetectable SCCA expression, had virtually no effect on IL-6 production. ( d ) CFPAC-1, L3.6 and HPAF-II cells were injected into the flanks of athymic nude mice and monitored for tumour growth; n =5. Representative images of tumour and the tumour growth curve±s.e.m. are shown; scale bar, 1 cm. * P <0.05, ** P <0.01, *** P <0.001 by t -test. Full size image In this study, we show that the endogenous serine/cysteine proteinase inhibitor SCCA is upregulated on activation of oncogenic Ras, in a manner that is dependent on hyper-active MAPK signalling and the ETS transcription factor PEA3. Downstream of oncogenic Ras, SCCA promotes activation of NF-κB signalling and cytokine production by blocking protein turnover and inducing the UPR. Our study implicates SCCA as a direct link between oncogenic Ras mutation, NF-κB activation and cytokine production. While it has been clearly demonstrated that the mutant Ras can activate NF-κB and induce inflammatory cytokine production in various settings, the underlying molecular mechanism has remained elusive. In numerous settings, inflammatory cytokine production has been attributed to oncogene-induced senescence that is associated with excess production of reactive oxygen species and subsequent DNA damage or loss of p53 (refs 6 , 27 ). We found that oncogenic Ras upregulates SCCA to promote cytokine production, whereas SCCA is not upregulated in the setting of drug-induced and replicative senescence. These results suggest that the secretory response seen in cells with oncogenic Ras mutations may be distinct from SASP induced by DNA damage or loss of p53. Although the physiological significance of Ras-induced cellular senescence remains an open topic, our results show that Ras can induce SCCA expression in cells where Ras does not induce senescence ( Fig. 1f ). Furthermore, we found that SCCA-dependent cytokine production occurs in human cells expressing endogenous level of mutant Ras ( Fig. 8 ) and this provides a mechanism that uncouples cellular senescence from inflammatory cytokine production on Ras activation. Importantly, our study shows that the incidence of SCCA positivity within PanIN lesions and PDAC increases with disease progression ( Fig. 7e ). Therefore, monitoring SCCA levels may become an attractive diagnostic tool in pancreatic cancer patients, as the levels of SCCA have been used in numerous studies to successfully predict disease stage and response to therapy [16] , [17] , [18] . Our work uncovers SCCA as a critical mediator of Ras-induced UPR. Until now, SCCA’s involvement in cancer was largely attributed to its protective role against lysosomal permeability that leads to unscheduled activation of lysosomal proteases [29] , [39] . We have previously reported that, through its protease inhibitory activity, SCCA leads to a decrease in both lysosomal and proteasomal protein turnover and elicits a non-lethal level of ER stress response [29] . It remains to be determined how SCCA mechanistically suppresses protein turnover, and whether other functions of SCCA such as its possible role in the nucleus contribute to increased UPR. Nevertheless, here we show that SCCA-mediated UPR plays a critical role in the context of oncogenic Ras mutation. Enhanced UPR has been well implicated in cancer, largely owing to the highly proliferative status of cancer cells and their encounter of growth limiting conditions such as nutrient deprivation and hypoxia [40] , [41] . Targeting the enhanced UPR of cancer cells remains an attractive therapeutic option, although the precise prediction of sensitivity has been difficult. Consistent with this notion, tumours driven by the mutant Ras have been shown to be susceptible to proteotoxic therapies [42] . Our current work showing that SCCA expression is stimulated by oncogenic Ras and plays an essential role in Ras-induced ER stress response, together with our previous report demonstrating SCCA sensitizes cells to proteotoxic stress [29] , suggest that SCCA may be a valuable predictor of response to proteotoxic agents in tumours harbouring oncogenic Ras. The contribution of the tumour stroma and inflammation to tumour development and progression, especially in pancreatic and colorectal cancer, is well accepted [43] , [44] . While NF-κB signalling has been shown to mediate the SASP response [26] , it is critical for the development of Ras-driven lung adenocarcinoma [45] . The pro-tumorigenic role of SCCA mediating NF-κB activation and inflammatory cytokine production is consistent with these reports. This adds a new pro-tumour mechanism of SCCA in addition to its well-documented anti-cell death function [15] , [46] , [47] , [48] , [49] . In a parallel study, we find that ectopic expression of SCCA can independently promote the transformation of the non-tumorigenic mammary epithelial cell line MCF10A (Sheshadri et al. , in preparation). As numerous studies utilizing anti-inflammatories to target the tumour microenvironment have shown great promise in the treatment of malignancies [50] , [51] , the ability of SCCA to promote cytokine production and tumorigenesis suggests a therapeutic value of targeting its protease inhibitory activity. Cell lines and culture 293T, IMR90, BJ, HT-29, Caco-2, HeLa, AsPC-1, Capan-1, Capan-2, CFPAC-1, HPAF-II, L3.6, PANC-1, PL45 and S2-013 cells were cultured according to ATCC recommendations. 293T, HeLa, PANC-1, PL45 and S2-013 cells were cultured in DMEM supplemented with 10% FBS (HyClone). IMR90, BJ and HPAF-II cells were cultured in MEM supplemented with 10% FBS. HT-29 and Capan-2 cells were cultured in McCoy’s 5a supplemented with 10% FBS. Caco-2 cells were cultured in MEM supplemented with 20% FBS. AsPC-1 and L3.6 cells were cultured in RPMI supplemented with 10% FBS. Capan-1 cells were cultured in Iscove’s supplemented with 20% FBS. CFPAC-1 cells were cultured in Iscove’s supplemented with 10% FBS. All media were supplemented with 100 units per ml penicillin and 100 μg ml −1 streptomycin (Invitrogen). Plasmids and reagents Retroviral expression vectors for WZL-hygro and WZL-HRas V12 were a kind gift of Dr Alea Mills at Cold Spring Harbor Laboratory [21] . pBABE-puro and pBABE-KRas V12 were a kind gift of Dr Scott Lowe at Memorial Sloan-Kettering Cancer Institute. pBABE-NRas Q61 was purchased from Addgene (Dr Channing Der; Plasmid 12543) [52] . pLNCX-ER:HRas V12 was a kind gift of Dr Masashi Narita at University of Cambridge [20] . pcDNA3-FLAG-ERK2-WT and pcDNA3-FLAG-ERK2-T138A (DN) were a kind gift of Dr Scott Eblen at the Medical University of South Carolina [53] . pcDNA3-PEA3-WT and pcDNA3-PEA3-K123R (MUT) were a kind gift of Dr Andrew Sharrocks at the University of Manchester [24] . Human XBP1s was cloned by RT-PCR from total RNA from IMR90 cells. Primers used were as follows, forward with HindIII restriction and FLAG tag: 5′-AAGCTTATGGATTACAAGGATGACGATGACAAGTGGTGGTGGCAGCCGCGCCGAACCC-3′ and reverse primer with HindIII restriction site: 5′-AAGCTTTTAGACACTAATCAGCTGGGGAAAG-3′. The RT-PCR product was digested with HindIII and ligated into the pLPC retroviral expression vector. All shRNA lentiviral constructs were in the pLKO (Sigma) backbone. shRNA targeting sequences used are shGFP: 5′-TACAACAGCCACAACGTCTAT-3′; shScramble: 5′-CAACAAGATGAAGAGCACCAA-3′; shSCCA#1: 5′-GCACAACAGATTAAGAAGGTT-3′; shSCCA#2: 5′-CCGCTGTAGTAGGGATTCGGAT-3′; shPEA3: 5′-GCTCCGATACTATTATGAGAA-3′; shATF6: 5′-GCAGCAACCAATTATCAGTTT-3′; shXBP1: 5′-GCCTGTCTGTACTTCCATTCAA-3′; shKRas: 5′-CAGTTGAGACCTTCTAATTGG-3′. Bay-11-7082 (B5556), 4-hydroxytamoxifen (H7904) and crystal violet (C0775) were purchased from Sigma. U0126 (V1121) was purchased from Promega. AKT inhibitor VIII (124018) was purchased from Calbiochem. TNFα (210-TA) was purchased from R&D Systems. X-gal (15520-018) was purchased from Invitrogen. Etoposide (8154-1) was purchased from Clontech. DNA transfection and viral infection Both retrovirus and shRNA lentivirus were generated in 293T cells. In brief, 293T were transfected by Lipofectamine 2000 (Invitrogen) with the plasmid of interest, packaging plasmid, and a plasmid encoding for the VSV-G envelope protein. Forty-eight and seventy-two hours after initial transfection, viral supernatant was collected, filtered, supplemented with polybrene (10 μg ml −1 ) and used to infect target cells. Forty-eight hours after last infection, cells were selected with appropriate antibiotics. IMR90 cells were selected for 2 days with 100 μg ml −1 of hygromycin, 2 μg ml −1 of puromycin or 1.75 mg ml −1 of G418. HeLa and L3.6 cells were selected with 0.5 μg ml −1 of puromycin for 2 days. Caco-2, Capan-1, CFPAC-1 and PANC-1 cells were selected with 1.0 μg ml −1 of puromycin for 3 days. Immunoblot analysis Cell lysates were prepared in RIPA buffer (1% sodium deoxycholate, 0.1% SDS, 1% Triton X-100, 0.01 M Tris pH 8.0, 0.14 M NaCl). Protein expression was examined by western blotting using antibodies against SCCA1/2 (FL-390; Santa Cruz; 1:1,000), Ras (Clone Ras10; Millipore; 1:10,000), p21 (C-19; Santa Cruz; 1:500), ERK1/2 (4,695; Cell Signaling; 1:10,000), P-ERK1/2 (4,370; Cell Signaling; 1:2;000), Akt (9,272; Cell Signaling; 1;2,000), P-Akt (4,058; Cell Signaling; 1:2,000), P-RelA/p65 (3,031; Cell Signaling; 1;1,000), RelA/p65 (F-6; Santa Cruz; 1:2,000), ATF6 (F-7; Santa Cruz; 1:500), XBP1 (M-186; Santa Cruz; 1:500), Ubiquitin (P4D1; Covance; 1:1,000) and β-tubulin (Sigma; 1:10,000). All primary antibodies were incubated overnight at 4 °C. Horseradish peroxidase or Alexafluor-conjugated goat anti-rabbit (Rockland) or goat anti-mouse (Rockland) antibodies were used as secondary antibodies (1:2,000). Western blots were developed using an ECL detection kit (Thermo Scientific) or an Odyssey Imager (LI-COR). Full scans of uncropped blots can be found in Supplementary Figs 9,10 . Gene expression analysis and quantitative PCR Total RNA was isolated and purified using the RNeasy kit (Qiagen). cDNA was obtained by reverse transcribing 1–2 μg of total RNA using SuperscriptIII Reverse Transcriptase (Invitrogen) and used for qPCR. qPCR reactions were performed in triplicate using SYBR Green reagents (Quanta Biosciences) on a StepOnePlus (Life Technologies). GAPDH was used as an endogenous control. All results were normalized to GAPDH. Primer sets used are: GAPDH: 5′-AAGGTCGGAGTCAACGGATTT G-3′ and 5′-CCATGGGTGGAATCATATTGGAA-3′; SCCA1: 5′-AGCCGCGGTCTCGTGC-3′ and 5′-GGCAGCTGCAGCTTCTG-3′; SCCA2: 5′-AGCCACGGTCTCTCAG-3′ and 5-GCAGCTGCAGCTTCCA-3′; Serpinb3a: 5′-CATTTGTTTGCTGAAGCCACTAC-3′ and 5′-CATGTTCGAAATCCAGTGATTCC-3′; Serpinb3b: 5′-ATTCGTTTTCATGCAGCTGATGT-3′ and 5′-GAAAGCTGAAGTTAAATTTGTTCG-3′; PEA3: 5′-GGACTTCGCCTACGACTCAG-3′ and 5′-CGCAGAGGTTTCTCATAGCC-3′; IL-6: 5′-TCCACAAGCGCCTTCGGTCCA3′ and 5′-AGGGCTGAGATGCCGTCGAGGA-3′; IL-8: 5′-AAGGAAAACTGGGTGCAGAG-3′ and 5′-ATTGCATCTGGCAACCCTAC-3′; CXCL1: 5′-CACCCCAAGAACATCCAAAG-3′ and 5′-TAACTATGGGGGATGCAGGA-3′; G-CSF: 5′-ACTACAAGCAGCACTGCCCT-3′ and 5′-AGCAGTCAAAGGGGATGACA-3′; GM-CSF: 5′-CAAGTGAGGAAGATCCAGGG-3′; and 5′-AGAGAGTGTCCGAGCAGCAC-3′. Cytokine array Cells were washed once with PBS and incubated for 8 h with fresh media. Supernatant was collected, cleared by centrifugation and used immediately. The amount of supernatant used was normalized to cell number and used with the human cytokine array kit (R&D Systems). IRDye 800CW Streptavidin (Rockland) was used as secondary (1:2,000) and arrays were imaged and quantified on an Odyssey Imager. Senescence assays Senescence was induced by oncogenic Ras, etoposide (100 μM, 48 h), H 2 O 2 (100 μM, 1 h) or long-term passaging (replicative senescence). All cells were analysed 7 days post-selection or post-treatment. For SA-β-gal staining, cells were fixed in 2% formaldehyde, 0.2% glutaraldehyde in PBS for 15 min and stained (150 mM NaCl, 2 mM MgCl 2 , 5 mM K 3 Fe(CN) 6 , 5 mM K 4 Fe(CN) 6 , 40 mM NaPi, pH 6.0, 1 μg ml −1 X-Gal) overnight at 37 °C. For BrdU staining, cells were cultured with BrdU (10 nM) for 6 h, fixed with acid ethanol (90% ethanol, 5% acetic acid, 5% H 2 O) for 30 min at room temperature. Cells were then washed once with PBS, incubated with 2 M HCl for 20 min, 0.1 M sodium borate, pH 8.5 for 2 min and washed once with PBS. Cells were blocked in 10% bovine serum albumin (BSA) in PBS for 1 h at room temperature and incubated with anti-BrdU (BD Pharmingen, 1:500 in 5% BSA in 0.1% PBS-tween) overnight at 4 °C. Cells were washed, incubated with anti-mouse Alexa-594 (1:500) for 1 h at room temperature, washed, co-stained with 4',6-diamidino-2-phenylindole (DAPI) and mounted. NF-κB luciferase activity assay NF-κB activity was determined by using an NF-κB luciferase reporter construct where the luciferase gene is under control of the IL-6 promoter and internal control plasmid pCMV-RL using a dual-luciferase reporter system (Promega). Cells were plated 24 h before transfection at 5 × 10 4 cells per well of 24-well plate. NF-κB-luciferase vector (250 ng) and 100 ng pCMV-RL were used for transfection. Twenty-four hours post transfection, cells were washed with PBS and lysed in 100 μl passive lysis buffer for 10 min. Luciferase activity was determined following the manufacturer’s recommended protocol with a SpectraMax M5 Microplate Reader. The ratios of firefly luciferase versus renilla luciferase are used as relative luciferase activities. TCGA analysis TCGA human colorectal cancer (study abbreviation: COADREAD) data were downloaded from Broad Institute’s Genome Data Analysis Center (GDAC). Standard data of somatic mutations (Mutation_Packager_Calls_Level_3) and RNA expression (Merge_transcriptome__agilentg4502a_07_3__unc_edu__Level_3__unc_lowess_normalization _gene_level__data.Level_3) were used. There were 207 human colorectal tumours that have both somatic mutation and mRNA expression data available. KRas was mutated in 87 out of the 207 samples. SCCA mRNA expression level was compared between the groups with wild-type and mutant KRas. Immunohistochemistry Tissue microarrays came from the Vanderbilt GI SPORE Tissue Core. Distribution and the use of all human samples were approved by the Institutional Review Boards of Vanderbilt University Medical Center and Stony Brook University, and samples were obtained with informed consent. IHC was performed on a Ventana XT (Tucson, AZ, USA) autostainer, according to the manufacturer’s directions. Tissue microarray analysis Damaged core spots and those that did not contain cancerous tissue were eliminated from scoring. The sections were scored independently by two evaluators blinded to the clinical status of the patients. Samples were scored as previously described [10] . In brief, samples were scored as percent of tumour cells with SCCA or IL-6 expression: 0, no expression; 1, <10%; 2, 10–50%; 3, >50%. For SCCA, a score ≥1 was considered positive. For IL-6, 0, negative; 1, weak; 2, moderate; 3, strong. Xenograft tumour experiments Male athymic nude mice, 6- to 8 weeks old, were obtained from Taconic Farms. Mice were housed and monitored at the Division of Laboratory Animal Resources at Stony Brook University. All experimental procedures and protocols were approved by the Stony Brook University institutional animal care and use committee (IACUC). Tumours were established by resuspending 1 × 10 6 tumour cells in 100 μl PBS and injecting the cells into the mid-flanks of mice using a 26-gauge needle. For each tumour, the tumour length ( l ) and width ( w ) was measured every 4–5 days with an electronic caliper. Tumour volume ( v ) was calculated using the formula v =( l × w 2 )/2 and plotted in mm 3 . Statistical analysis Statistical analyses were performed with GraphPad Prism (Graphpad Software Inc). For gene expression, luciferase activity and xenograft tumour growth significance was calculated with t -tests. χ 2 -tests were used to assess statistical significance of various categorical clinical features between SCCA-negative and SCCA-positive samples. For the TCGA colorectal cancer data analysis, Wilcoxon Rank Sum test was performed. For all tests, P -values were considered statistically significant when <0.05. How to cite this article: Catanzaro, J. M. et al. Oncogenic Ras induces inflammatory cytokine production by upregulating the squamous cell carcinoma antigens SerpinB3/B4. Nat. Commun. 5:3729 doi: 10.1038/ncomms4729 (2014).